Reduced selection and accumulation of deleterious mutations in genes exclusively expressed in men Sex-limited selection can moderate the elimination of deleterious mutations from the population and contribute to the high prevalence of common human diseases. Accordingly, deleterious mutations in autosomal genes that are exclusively expressed in only one of the sexes undergo sex-limited selection and can reach higher frequencies than mutations similarly selected in both sexes. Here we show that the number of deleterious SNPs in genes exclusively expressed in men is twofold higher than in genes that are selected in both sexes. Additional analyses suggest that the increased number of damaging mutations we found in male-specific genes is due to reduced selection in females. These results are noteworthy since many of these male-specific genes are known to be crucial for male reproduction, and are thus likely to be under strong purifying selection. We suggest that inheritance of male-infertility-causative mutations through unaffected female lineages contributes to the high incidence of male infertility. Many common diseases have a strong genetic basis [1] . Moreover, the common disease–common variant hypothesis posits that common, disease-associated alleles affect the prevalence of most common diseases [2] , [3] . These findings led to the question of how deleterious mutations accumulate in the human population when they are expected to be under strong purifying selection. Several explanations for the relative prevalence of deleterious mutations, in general, are well established. Mutation-selection balance posits that the equilibrium frequency of alleles largely depends on the balance between the mutation rate and selection pressure [4] . Hence, elevated mutation rates of an allele can lead to higher equilibrium frequencies even if the selection pressure on the allele is the same as on other alleles. The heterozygote advantage is suggested in cases where recessive deleterious mutations become beneficial in the heterozygote status, for example, in sickle cell anaemia [5] . It is also possible that genotypes that were beneficial in the past and under different environmental conditions are currently harmful, as suggested in the ‘thrifty gene’ theory [6] . The sense of smell is a related case of reduced dependency on a previously essential trait as reflected by olfactory receptor gene loss in primates and allele loss in human populations [7] . Besides these explanations, disease parameters such as age of onset and severity undergo different selection pressures [8] that might affect the tendency of the causative mutations to accumulate in the population. Finally, non-adaptive processes, such as bottlenecks and fluctuation in population sizes over evolutionary time, enable slightly deleterious mutants to reach high frequencies because of founder effects [9] and can also explain the establishment of severe mutations in the population [10] . Such explanations do not account well for lethal and sterility-causing mutations, which are not expected to accumulate in the population since they directly reduce the number of the individual’s progeny [11] . However, human infertility has a strong genetic basis and being a very common disorder seems to be a paradox [12] , [13] , [14] . Differential selection because of sexual dimorphisms was also suggested and modelled as a mechanism that contributes to the propagation of deleterious mutations in the population [15] , [16] . This mechanism specifically suggested and later was shown to contribute to the propagation of deleterious mutations in the maternally inherited mitochondrial DNA (mtDNA) [17] . Differential selection occurs since mutations in mtDNA that solely affect sperm biogenesis can only be selected in males but the mtDNA is only inherited through females. Autosomal and X-linked genes that have sex-limited expression are also expected to undergo differential selection, leading to higher number and elevated frequencies of deleterious mutations in these genes, as compared with genes that are similarly selected in both sexes. This was demonstrated on the bcd maternally expressed gene that was shown to have twice as many non-synonymous, but not synonymous, mutations than its zygotic expressed paralogue zen [18] , [19] . Genes that are exclusively expressed in human testes are sex-limited and are therefore expected to undergo differential selection. Deleterious mutations in these genes are thus expected to accumulate at higher frequencies relative to mutations with similar phenotypic effect in both sexes, since they are not selected in about half of the population. In this work, we examine the propagation of deleterious mutations in autosomal and X-linked genes that are exclusively expressed in human testes and are thus sex-limited. Deleterious mutations in these genes potentially reduce individual fitness, specifically male reproductive success. A computational screen identified genes with different male-specificity expression levels, and genes with corresponding expression patterns in other tissues, biochemical functions and biological processes. The propagation of deleterious mutations in the human population was computed for the identified gene groups and for random gene sets. Here we find that autosomal genes exclusively expressed in men harbour twofold more deleterious mutations than genes expressed in both sexes, and that this is likely due to lack of selection in women. Our findings are consistent with the hypothesis for reduced selection efficiency on non-Y-linked sex-limited genes (that is, genes carried by both sexes but solely expressed in males or females). We discuss the implications of our findings for human variation, genetic fertility disorders and sexual dimorphic genetic traits. Identifying male-specific genes and control groups To test for reduced selection on testis-exclusive genes because of differential selection, we first identified such human genes and genes for appropriate controls. Y-linked genes were omitted from the analysis since they are not present in females and have only one copy in males, and are thus irrelevant to the reduced selection hypothesis. Using expression data from 79 diverse normal tissues [20] we found 95 testis-exclusive genes. In the same manner we identified 13 non-testes human tissues with sufficient exclusive gene expression data (465 genes; Supplementary Tables 1–15 ). Data did not include a sufficient number of female-specific tissues for analysis (for example, we could only identify one ovary-exclusive gene). 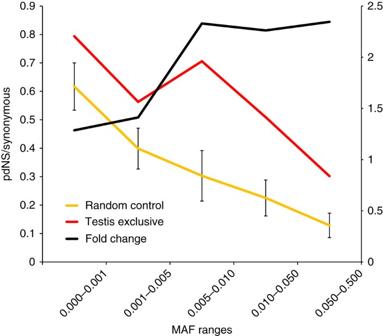Figure 1: pdNS accumulation tendency is significantly higher in testis-exclusive genes compared with random control. Accumulation of pdNS normalized by synonymous mutations (leftyaxis) in different MAF ranges (xaxis) in the testis-exclusive gene group (red line) and in 10,000 sets of randomly picked genes (yellow line). The black line represents the increase change between the testis-exclusive group and the random sets (rightyaxis). The left to right MAFs binsPvalues after FDR correction are 0.022, 0.022, 0.001, 0.0005 and 0.001, respectively,N=10,000 sets of 95 genes. The error bars represent the s.d. of the 10,000 sets for each MAF bin. Additional control gene groups were non-testes paralogues of the testis-exclusive genes (216 genes; Supplementary Table 16 ), non-testes male reproduction genes (372 genes; Supplementary Table17 ), testes highly specific genes (72 genes; Supplementary Table 18 ) and 10,000 sets of 95 randomly selected human genes (corresponding to the size of the testis-exclusive gene group). Gene variation analyses The ‘1000 Genomes’ project [21] phase-1 data were used to assess the numbers of predicted deleterious non-synonymous (pdNS) single-nucleotide length polymorphisms (SNPs), nonsense (stop-gain) SNPs and synonymous SNPs, in each gene of the examined groups and sets. We also retrieved the SNP’s minor allele frequencies in the population (MAF), and the evolutionary conservation scores [22] of all analysed variations. Non-synonymous mutations are heterogeneous, with some of the mutations functional and others neutral or slightly functional [23] . We therefore used pdNS mutations, rather than all non-synonymous mutations, since they are more likely to cause functional alterations in proteins, and are thus more likely to be under selection. This is also reflected in the purifying selection rate for each mutation type ( Supplementary Fig. 1 ). The pdNS accumulation tendencies were calculated to be the number of pdNS SNPs in increasing MAF ranges, normalized by the number of synonymous SNPs in the same MAF range. The 95 testis-exclusive genes are significantly enriched in male fertility genes and disorders ( Table 1 ). Genetic studies of male sterility identified the causative mutation in 22 of these genes [12] . Deleterious mutations in the testis-exclusive genes are therefore likely to be under strong negative selection. Table 1 Gene annotation term (DAVID) and disorder (GeneDecks) enrichment of the testis-exclusive gene group. Full size table Testes-exclusive genes have more deleterious mutations Natural gene variants are of different frequencies, with most of the variation due to alleles with rare to low MAF [23] . However, selection is not expected to have a significant effect on the propagation of rare variations. These variations are predominantly new, while selection is mainly a long-term process. In addition, most phenotypes are due to allele and gene interplay, and thus are highly unlikely (except in inbreeding) for rare variations, for example, recessive and epistatic models of inheritance [23] , [24] . We thus compared the normalized numbers of pdNS mutations for different MAF ranges in the ‘1000 Genomes’ project between the 95 testis-exclusive genes and a random control (10,000 sets of 95 randomly chosen genes from all non-Y-linked protein-coding genes in Ensembl version 69). The ratio of the numbers is always higher for the testis-exclusive gene group. For the rarest mutations (MAF<0.001) the testis-exclusive gene group has significant 1.3 higher pdNS number (randomization test, N =10,000 sets of 95 genes, false discovery rate (FDR) correction, P =0.02). However, the number of pdNS mutations in the testis-exclusive gene group becomes highly significant and more than twofold higher for MAF ranges of 0.005 or above (randomization test and FDR correction, N =10,000 sets of 95 genes, 0.01≥MAF≥0.005, P =0.001; MAF≥0.005 P <0.0001; Fig. 1 ). We thus used a threshold of MAF≥0.005 (0.5%) since SNPs below that value are subject to reduced efficient selection [23] . Three of the 95 testis-exclusive genes are X-linked and might have different selection constraints. However, the same results are observed when these three testis-exclusive and X-linked genes are omitted from the testis-exclusive gene group ( Supplementary Fig. 2 ). None of the 10,000 random-control gene sets had an equal or higher number of pdNS mutations than the testis-exclusive gene group for MAF≥0.005. We also note that the testis-exclusive and random sets show reduced normalized pdNS mutation numbers for higher MAF, indicating that the pdNS mutations are eliminated from the population under purifying selection, and thus are probably deleterious. We performed the same analyses for stop-gain mutations that are expected to be highly deleterious since they truncate the protein encoded by the gene ( Supplementary Fig. 1 ). The testis-exclusive gene group was found to accumulate significantly more stop-gain mutations (randomization test, N =10,000 sets of 95 genes, P =0.005 for MAF≥0.005) relative to 10,000 sets of 95 random genes ( Supplementary Fig. 3 ). Figure 1: pdNS accumulation tendency is significantly higher in testis-exclusive genes compared with random control. Accumulation of pdNS normalized by synonymous mutations (left y axis) in different MAF ranges ( x axis) in the testis-exclusive gene group (red line) and in 10,000 sets of randomly picked genes (yellow line). The black line represents the increase change between the testis-exclusive group and the random sets (right y axis). The left to right MAFs bins P values after FDR correction are 0.022, 0.022, 0.001, 0.0005 and 0.001, respectively, N =10,000 sets of 95 genes. The error bars represent the s.d. of the 10,000 sets for each MAF bin. Full size image Comparing testis-exclusive to other tissue-exclusive genes To determine whether deleterious mutations in the testis-exclusive genes tend to accumulate in the population twofold higher than by chance is due to their being sex-limited or to other properties of these genes, we performed several control analyses. First, the high tendency to accumulate deleterious mutations may result from the testis-exclusive genes being expressed in only a single tissue [25] , [26] . To address this possibility we used the 13 groups of exclusively expressed genes from diverse non-testes tissues ( Supplementary Tables 1, 3–15 ). Each of the tissue-exclusive gene groups (testis-exclusive and 13 others) was compared with all other tissue-exclusive genes. Only the testis-exclusive gene group deviated from all other tissue-exclusive genes, having a significantly higher tendency to accumulate pdNS (one-tailed χ 2 and FDR correction, N testes =95, N other tissues =465, P =1.60E-04), and to accumulate stop-gain mutations (one-tailed binomial exact test and FDR correction, N testes =95, N other-tissues =465, P =5.00E-02; see Fig. 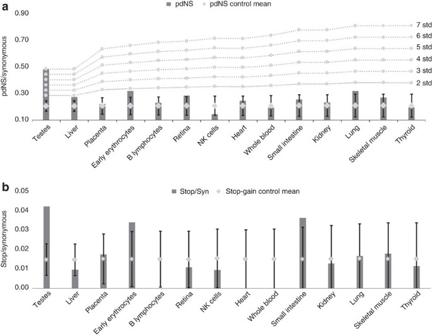Figure 2: Tissue-exclusive group pdNS and stop-gain mutation accumulation tendencies. Accumulation of pdNS (a) and stop-gain (b) mutations with MAF≥0.005 normalized by corresponding synonymous mutations (yaxis) in diverse tissue-exclusive gene groups (xaxis). Diamonds show the mean values expected by chance, error bars show ±1 s.d., and dotted lines show 2–7 s.d. values. The mean and s.d. were calculated for each tissue-exclusive group by a randomization test. Only the testis-exclusive gene group (left-most bar) has significantly higher pdNS (6.9 s.d.) and stop-gain (3.1 s.d.) values,Ntestes=95. 2 and Table 2 ). Figure 2: Tissue-exclusive group pdNS and stop-gain mutation accumulation tendencies. Accumulation of pdNS ( a ) and stop-gain ( b ) mutations with MAF≥0.005 normalized by corresponding synonymous mutations ( y axis) in diverse tissue-exclusive gene groups ( x axis). Diamonds show the mean values expected by chance, error bars show ±1 s.d., and dotted lines show 2–7 s.d. values. The mean and s.d. were calculated for each tissue-exclusive group by a randomization test. Only the testis-exclusive gene group (left-most bar) has significantly higher pdNS (6.9 s.d.) and stop-gain (3.1 s.d.) values, N testes =95. Full size image Table 2 Deviations of each tissue-exclusive gene group from all other tissue-exclusive groups. Full size table Nevertheless, tissue specificity might still partially contribute to the high numbers of pdNS and stop-gain mutations relative to those expected by chance. This was tested by comparing the number of deleterious mutations of each tissue-exclusive gene group to 10,000 random-control gene sets, for MAF≥0.005. The number of genes in each set was equal to that of the examined group size. 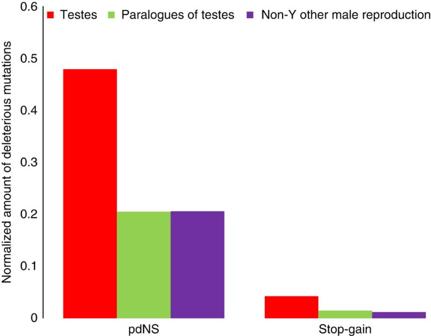Figure 3: pdNS and stop-gain accumulation tendencies are significantly higher in testis-exclusive genes compared with paralogues-of-testes and non-testes male reproduction gene groups. Accumulation of pdNS and stop-gain mutations normalized by synonymous mutations (yaxis) for MAF≥0.005 in the testis-exclusive gene group (red bar),N=95, the paralogues of the testis-exclusive gene group (green bar),N=216, and the non-Y-linked non-testis-exclusive male reproduction gene group (purple bar),N=372. None of the 13 non-testes tissue-exclusive gene groups were found to have a significantly higher number of pdNS or stop-gain mutations than expected by chance (randomization test, FDR correction, sample sizes are listed in Table 3 and in Supplementary Table 1 , 0.35≤ P ≤1; Table 3 and Fig. 2 ). Altogether, the contribution of tissue specificity to the accumulation tendency of deleterious mutations in testis-exclusive genes cannot be discerned and is negligible at most. Table 3 Randomization tests for the non-testis tissue-exclusive gene groups. Full size table Comparing testis-exclusive genes to their paralogues The significantly higher numbers of pdNS and stop-gain mutations in testis-exclusive genes might also be due to the biochemical functions of the gene products or to the male reproduction biological process they function in. This possibility was addressed by repeating the same analyses on the paralogues of the testis-exclusive genes (genes that should have relatively similar cellular and biochemical functions in other tissues), and on non-testis-exclusive male reproduction genes omitting Y-linked genes. Of the 95 testis-exclusive genes we found 45 to have several paralogues, 14 to have a single paralogue and 36 with no paralogues. A significant ~2.3-fold higher tendency to accumulate pdNS and stop-gain mutations for MAF≥0.005 was observed in testis-exclusive genes relative to their non-testes paralogues (one-tailed χ 2 , FDR correction, N testes =95, N paralogues =216, P =2.08E−06 and P =0.03, respectively), and to the non-testis-exclusive male reproduction genes (one-tailed χ 2 , FDR correction, N testes =95, N male reproduction =372, P =1.95E−05 and P =0.03, respectively; Fig. 3 ). The high pdNS accumulation tendency of the testis-exclusive gene group remained highly significant after excluding the 36 testis-exclusive genes with no paralogues (one-tailed χ 2 , N testes =59, N paralogues =216, P =7E−8). Figure 3: pdNS and stop-gain accumulation tendencies are significantly higher in testis-exclusive genes compared with paralogues-of-testes and non-testes male reproduction gene groups. Accumulation of pdNS and stop-gain mutations normalized by synonymous mutations ( y axis) for MAF≥0.005 in the testis-exclusive gene group (red bar), N =95, the paralogues of the testis-exclusive gene group (green bar), N =216, and the non-Y-linked non-testis-exclusive male reproduction gene group (purple bar), N =372. Full size image Comparing testis-exclusive to testes highly specific genes On the basis of the reduced selection hypothesis, one could expect that the increased numbers of pdNS and stop-gain mutations in testis-exclusive genes are due to their lack of expression in female lineages. If so, we expected to find the increased tendencies of pdNS and stop-gain mutations in direct relation to the gene’s male expression specificity. Using the same measure of tissue-specific expression, we identified (for the testes and for other tissues) hundreds of genes with reduced levels of tissue-specific expression. The reduced tissue specificity levels vary from exclusive expression in one tissue to highly specific expression in a single tissue ( Supplementary Table 18 ) to solely nonspecific expression ( Fig. 4 ). The specificity level was measured quantitatively using a correlation coefficient (Methods). Qualitatively, ‘exclusive expression’ is expression in only one tissue, and ‘highly specific expression’ is typically a major expression in one tissue with a minor expression in one or two other tissues. Analysing gene groups with different tissue specificity expression levels we find a significant reduction in the accumulation of pdNS and stop-gain mutations (one-tailed χ 2 , MAF≥0.001, N exclusive =95, N highly specific =72; P =0.01, P =0.03, respectively) in genes that are highly specific to the testes but have minor expression in at least one other non-sex-specific tissue, in comparison with the testis-exclusive genes. No significant differences were found between exclusive genes and highly specific genes in non-testes tissue groups ( Fig. 4 ). 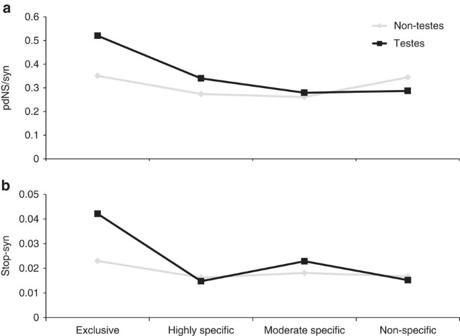Figure 4: pdNS and stop-gain mutation accumulation tendency is significantly higher in testis-exclusive genes compared with genes with reduced testis specificity. Accumulation of pdNS (a) and stop-gain (b) mutations with MAF≥0.001 in gene groups with differing expression specificity to testis (black squares) and non-testis tissues (light-grey diamonds). The testis-exclusive gene group (left-most black square) has a significantly higher pdNS (a, one-tailedχ2test,Nexclusive=95,Nhighly specific=72,P=0.01) and stop-gain (b, one-tailedχ2test,Nexclusive=95,Nhighly specific=72,P=0.03) accumulation tendencies relative to highly testis-specific genes (overexpressed in the testes with minor expression in other one or two non-sex-specific tissues). ‘Exclusive’ expression corresponds to correlation values of 1.0≥r>0.95 with an exclusive testis-expression profile (mask), ‘highly specific’ corresponds to 0.75≥r>0.65, ‘moderate specific’ corresponds to 0.45≥r>0.35, and ‘nonspecific’ corresponds to 0.11≥r>0.09. Figure 4: pdNS and stop-gain mutation accumulation tendency is significantly higher in testis-exclusive genes compared with genes with reduced testis specificity. Accumulation of pdNS ( a ) and stop-gain ( b ) mutations with MAF≥0.001 in gene groups with differing expression specificity to testis (black squares) and non-testis tissues (light-grey diamonds). The testis-exclusive gene group (left-most black square) has a significantly higher pdNS ( a , one-tailed χ 2 test, N exclusive =95, N highly specific =72, P =0.01) and stop-gain ( b , one-tailed χ 2 test, N exclusive =95, N highly specific =72, P =0.03) accumulation tendencies relative to highly testis-specific genes (overexpressed in the testes with minor expression in other one or two non-sex-specific tissues). ‘Exclusive’ expression corresponds to correlation values of 1.0≥ r >0.95 with an exclusive testis-expression profile (mask), ‘highly specific’ corresponds to 0.75≥ r >0.65, ‘moderate specific’ corresponds to 0.45≥ r >0.35, and ‘nonspecific’ corresponds to 0.11≥ r >0.09. Full size image Selection efficiency analysis Finally, the likelihood of a gene to undergo specific mutations might be affected by its sequence composition and protein function (for example, because of specific sequences such as excess of methionine codons where every mutation is non-synonymous, or protein function such as extreme conservation where most mutations will be deleterious). Thus, the higher numbers of deleterious mutations in such genes could be independent of selection. To examine this possibility we directly assessed the efficiency of selection on pdNS versus other types of mutations. We compared the numbers of normalized mutations of rare (MAF<0.001) versus common (MAF>0.010) pdNS, stop-gain and predicted non-deleterious non-synonymous (non-pdNS) mutations. We found that the selection efficiency for both pdNS and stop-gain mutations was more than twofold higher in all controls relative to the testis-exclusive gene group ( Fig. 5 ). The other NS mutations (predicted non-deleterious) are likely to be more neutral and therefore are expected to undergo reduced selection regardless of their gene’s sex-expression pattern. Indeed, contrary to the deleterious mutations, only a slight difference in selection efficiency (1.2- to 1.5-fold change) was found for the other (predicted non-deleterious) NS mutations. 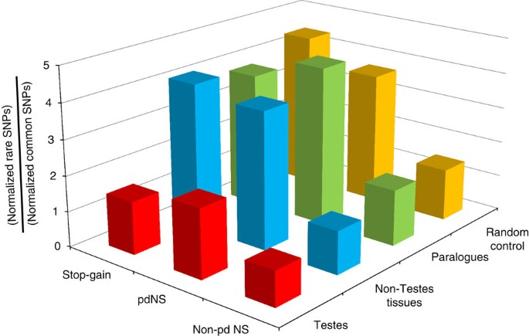Figure 5: Reduced selection efficiency on deleterious mutations in the testis-exclusive gene group. Selection efficiency for the testis-exclusive,N=95 (testes, red bar), non-testis tissue-exclusive expression,N=465 (non-testis tissues, blue bar), paralogues of testis-exclusive,N=216 (Paralogues, green bar) and the Random control gene sets,N=10,000 sets of 95 genes (yellow bar) is shown (xaxis) as the ratio of all rare (MAF≤0.001) to all common (MAF≥0.01) normalized mutations (yaxis), for non-pdNS, pdNS and stop-gain type mutations (zaxis). Figure 5: Reduced selection efficiency on deleterious mutations in the testis-exclusive gene group. Selection efficiency for the testis-exclusive, N =95 (testes, red bar), non-testis tissue-exclusive expression, N =465 (non-testis tissues, blue bar), paralogues of testis-exclusive, N =216 (Paralogues, green bar) and the Random control gene sets, N =10,000 sets of 95 genes (yellow bar) is shown ( x axis) as the ratio of all rare (MAF≤0.001) to all common (MAF≥0.01) normalized mutations ( y axis), for non-pdNS, pdNS and stop-gain type mutations ( z axis). Full size image Divergent and positive selection Many genes that mediate sexual reproduction, such as those involved in gamete recognition, are known to rapidly evolve, frequently under positive selection, during speciation [27] , [28] , [29] , [30] , [31] . We tested whether differences in the selection constraints during the divergence of testis-exclusive genes could explain their increased number of deleterious mutations. d N /d S analysis is a well-established measure of protein divergence, specifically between distant lineages with high d N /d S ratios (>1) indicating fast protein divergence, likely due to positive or relaxed selection constraints [32] , [33] . Thus, significant differences in d N /d S ratios of genes might indicate differences in their selection constraints. Comparing the mouse–human d N /d S distribution of the testis-exclusive group and all non-testes tissue-exclusive genes, we found no significant difference (two-tailed Kolmogorov–Smirnov (KS) test, N testes =95, N other tissues =465, P =0.26). This suggests that between human and mouse there are no overall significant differences in the testis-exclusive gene selection constraints in comparison with other tissue-exclusive genes. Nevertheless, the similarity in the d N /d S distributions does not rule out the possibility that some genes in the testis-exclusive gene group rapidly evolve under positive selection. Indeed, the literature reports that 5/95 genes of our testis-exclusive group underwent positive selection between human and chimpanzee ( ABHD1, TCP11 ) [28] , human and mice ( GAPDHS, ADAM2 ) [30] or both (PRM1). In addition, a recent variation analysis of whole exomes from ~2,500 human individuals reported 114 positively selected genes during human intraspecies evolution [23] . Of these only one gene ( CNTD1 ) is found in our testis-exclusive gene group. Removal of all these six positively selected genes from our testis-exclusive gene group did not affect the tendency to accumulate deleterious mutations ( Supplementary Fig. 2 ). Thus, 94/95 human testis-exclusive genes were not found to undergo positive selection in human intraspecies evolution, although another five of these genes did show positive selection during mammalian interspecies evolution. Finally, specific nucleotide positions within a gene can undergo selection regardless of the overall selection on the gene (for example, specific positions in a rapidly evolving gene can be extremely conserved and vice versa ). Since we found differences in the accumulation rate of specific mutations, that is, pdNS and stop-gain, we compared the pdNS gene positions’ evolutionary conservation [22] in different gene groups. No significant differences were found in the distribution of the evolutionary conservation scores for pdNS mutations of testis-exclusive genes relative to their paralogues, to non-testes tissue-exclusive genes, and to non-testis-exclusive male reproduction genes (two-tailed KS test and FDR correction, P =0.7; P =0.06; P =0.7, respectively; Fig. 6 ). 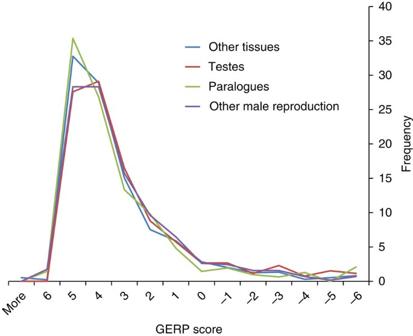Figure 6: Conservation analysis of the pdNS mutation sequence positions. Distributions of all pdNS-mutations sequence-position GERP scores (deficit in substitutions because of functional constraints22) for variation in the testis-exclusive gene group,N=95 (red line), in paralogues-of-testes gene group,N=216 (green triangles), in non-testis tissue gene group,N=465 (blue diamonds) and in non-testis-exclusive male reproduction genes,N=372 (grey squares) are shown. GERP score bins (between each consecutively shown value, with the left distal value all scores above 6) are on thexaxis, and their frequencies are on theyaxis. Figure 6: Conservation analysis of the pdNS mutation sequence positions. Distributions of all pdNS-mutations sequence-position GERP scores (deficit in substitutions because of functional constraints [22] ) for variation in the testis-exclusive gene group, N =95 (red line), in paralogues-of-testes gene group, N =216 (green triangles), in non-testis tissue gene group, N =465 (blue diamonds) and in non-testis-exclusive male reproduction genes, N =372 (grey squares) are shown. GERP score bins (between each consecutively shown value, with the left distal value all scores above 6) are on the x axis, and their frequencies are on the y axis. Full size image Differential selection because of sexual dimorphisms posits that genes that have different roles between males and females can have different selection constraints in each sex. In the extreme case, selection on mutations in such genes can be antagonistic, that is, positive in one sex and negative in the other. Therefore, mutations that can cause severe phenotypes in one sex can reach high frequencies in the population. We tested this hypothesis on testis-exclusive human genes, which by definition are sex-limited and are thus expected to be only selected in men. This hypothesis could explain the paradoxical inheritance of infertility-causing mutations and should be relevant to any species with different stable sexual morphs. Our results show that deleterious mutations in non-Y-linked testis-exclusive genes tend to accumulate in human populations more than deleterious mutations in other genes. This is most likely because of the sex-limited expression of testis-exclusive genes and the resulting absence of selection in females, and thus supports the hypothesis. We tested for accumulation of deleterious mutations in humans, which currently have publicly available genetic variation data for a large and representative population from the ‘1000 Genomes’ project [21] and on male-exclusive genes for which we found sufficient numbers of genes and proper controls. In principle, any genes that have a differential role between the sexes, with the most extreme case being the sex-exclusive genes, will be under differential selection that can lead to reduced selection efficiency (either positive or negative). In practice, to find such genes requires large-scale transcriptome sequencing in as many tissues and physiological and developmental conditions as feasible for each sex. While the technology for such an endeavour is currently available at steadily dropping costs, we could not at present find such public data. The ‘sex-exclusive genes’ were thus identified by their unique expression in sex-specific organs: that is, our testis-exclusive-expression gene group. Gene annotation analysis and literature searches show that human testis-exclusive genes are significantly enriched in male reproductive processes ( Table 1 ), and that mutations in some of these genes cause male infertility and sterility [12] . Thus, deleterious mutations in such genes are likely to be under extreme purifying selection. However, the testis-exclusive gene group we found showed a significantly higher accumulation tendency of pdNS mutations relative to random controls ( Figs 1 and 2 ). Although pdNS mutations are under purifying selection in both testis-exclusive and the random control groups ( Figs 1 and 5 ), the differences between these groups increase with increasing MAF and stabilize beyond a MAF value of 0.005 at about a twofold ratio. This reflects reduced selection efficiency on the testis-exclusive genes. Selection efficiency greatly depends on the effective population size and mutation frequencies [34] . Since mutations in testis-exclusive genes are selected only in about half of the population (that is, only in males), their effective population size is expected to be about half that of mutations in genes undergoing similar selection pressure in both sexes [18] , [19] . Thus, the twofold difference we observed might reflect the halving of the effective population size. In addition, the 0.005 MAF threshold we found might indirectly predict the effective population size in which the selection was predominant. Testes-exclusive genes are tissue-specific, and such genes were shown to evolve more rapidly during speciation than housekeeping genes [25] . This might result mainly from the tissue-specific genes being more adaptable due to fewer pleiotropic effects [26] . However, tissue specificity does not explain our findings since the testis-exclusive gene group had a significantly higher tendency to accumulate deleterious mutations than all other groups of tissue-exclusive genes ( Fig. 2 and Supplementary Fig. 4 ). Moreover, all other tissue-exclusive gene groups accumulated deleterious mutations as expected by chance. We also found a significant difference between testis-exclusive genes and testis-highly specific genes ( Fig. 4 ). Thus, even minor expression in non-testes tissue reduces the tendency to accumulate more deleterious mutations in genes that are predominantly expressed in the testes. This indicates that high testes expression specificity in itself is unlikely to be the cause for the higher accumulation tendency of deleterious mutations. Significant differences were also found when comparing the testis-exclusive genes to their paralogues and to non-testis-exclusive male reproduction genes ( Fig. 3 ), suggesting that the reduced selection is unrelated to the genes’ biochemical functions and biological process. To assess the accumulation tendencies of different mutation types (that is, pdNS, stop-gain, non-pdNS), we normalized the number of each mutation type with the number of synonymous mutations in every gene group. This normalization takes into account both the genes’ coding lengths and their mutation rates. In addition, this accounts for non-adaptive processes and stochastic events that similarly affect all types of mutations in the gene. However, genes might also have significantly different probabilities to undergo a specific type of mutation (for example, synonymous or deleterious mutations) because of their sequence composition or their protein function. This might result in spuriously high or low accumulation tendencies, regardless of selection. These possibilities were dismissed by selection efficiency analyses. Assuming that the occurrence of new mutations [35] and the likelihood for mutations of a certain type in a gene group do not change over time, the differences in the normalized numbers of rare to common mutations are expected to directly reflect the selection efficiency. We found about twofold higher selection efficiency on pdNS, and about 2.5-fold higher on stop-gain mutations in all control groups relative to the testis-exclusive genes ( Fig. 5 ). These findings are consistent with the testis-exclusive genes exposed to selection only half the time (that is, only when passing through men), relative to other genes. We also compared the selection efficiency of predicted non-deleterious non-synonymous mutations (non-pdNS) between the different gene groups. Non-pdNS mutations are those predicted to be benign by either Polyphen, SIFT or both methods, and are thus expected to be more neutral and less affected by selection than the pdNS mutations. Indeed, we found reduced differences in the selection efficiency on non-pdNS in testis-exclusive genes relative to controls, supporting the main concept of selection relaxation on deleterious mutation, and contrary to a general acceleration in testis-exclusive gene evolution ( Fig. 5 ). Finally, several studies have shown that some genes associated with reproduction in general, and specifically with male reproduction, tend to evolve more rapidly during speciation [27] , [28] , [29] , [30] , [31] . It is thus possible that accelerated evolution of genes involved in the reproductive process, as reflected by interspecies comparisons, could also be present within populations of a given species (intraspecies). However, our testis-exclusive gene group only included a few rapidly diverging or positively selected genes, whose removal from the group does not change its pdNS or stop-gain mutation tendencies. Furthermore, we did not find any significant differences between the testis and non-testis-exclusive genes d N /d S distribution. The conservation of the pdNS gene positions in testis-exclusive genes is also no different from that of the controls ( Fig. 6 ), indicating similar functional importance and evolution of the specific SNP sites. In addition, a recent work reported 114 rapidly evolving and positively selected genes in the human population but no enrichment of positively selected genes in male reproduction genes was reported [23] , and only a single gene of these was found in our testis-exclusive gene group. Thus, testis-exclusive genes are not undergoing rapid adaptive changes within humans, and rapid adaptive evolution, inter- or intraspecies, cannot explain our findings. Overall, the conservation and selection patterns of the testis-exclusive genes are no different than all other control groups we examined. Finally, genes involved in the immune response course were also reported to be positively selected during radiation of mammals [36] , [37] . We found no significant tendency to accumulate pdNS or stop-gain mutations in our two immune-response associated tissue-exclusive gene groups, that is, NK cells and the B lymphocytes. In this work we analysed autosomal and X-linked genes together, even though their selection constraints might differ for male-specific genes of these two types. Deleterious mutations on male-specific genes may be expected to accumulate more rapidly on X-linked genes, relative to autosomal genes, since females carry two alleles and males only one. Countering this is the probable stricter selection of such genes in males due to their hemizygous (single copy) state. We cannot examine how these two opposing forces affect the tendency to accumulate deleterious mutations in our data since we have found only three X-linked testis-exclusive genes. Removing these three genes from the other 95 male-exclusive genes did not change our findings on the accumulation of deleterious mutations in male testis-exclusive genes ( Supplementary Fig. 2 ). Taken together, our results show that deleterious mutations in male testis-exclusive genes tend to accumulate significantly more than expected from the overall accumulation mutation tendencies, from tissue-exclusive expression, from the function of these genes, and from the evolution of male reproduction genes. The increased tendency to accumulate deleterious mutations in male testis-exclusive genes is thus because of reduced purifying selection, most likely caused by their absence of expression in females. Many common human diseases and traits with significant impact on public health are sexually dimorphic or undergo different disease courses in the sexes. Examples include schizophrenia, Parkinson disease and colorectal cancer that are more common in men, and depression and autoimmune diseases that are more prevalent in females [38] , [39] , [40] , [41] , [42] , [43] . The vast majority of sexually dimorphic traits result from differential expression of genes present in both sexes. This implies that these genes will be subject to different selection levels in the two sexes, and might even be subject to conflicting selective pressures between the sexes [44] . Hence, it has also been shown in the fruit fly that mutations in genes with sex-biased expression have also sex-biased phenotypic consequences [45] . Another level of selection constraint could stem from the fact that most male gametes do not fertilize any eggs. Reduction in the number of successfully reproducing males was thus suggested to be more tolerable in the population than such a reduction in females. By this argument, male-specific genes are expected to be under less selection than female-specific genes [46] . We could not find sufficient numbers of female-specific genes to examine; however, we expect deleterious mutations in such genes to also accumulate more relative to equivalent genes with similar functional importance in both sexes. Identifying accumulation of deleterious mutations in female-specific genes and in additional male-specific genes (that is, not particular to sex-specific tissues) will reinforce our findings and interpretations. This is important since currently we cannot completely rule out that our findings stem from some unidentified property of genes that are exclusively expressed in the testes. We conclude that deleterious mutations in male testis-exclusive genes tend to accumulate in the human population in spite of the morbid phenotypes they are likely to cause, specifically in male reproduction processes. The more than twofold higher occurrence of such mutations in male-specific genes, relative to the other gene groups we tested in this work, is remarkable since these mutations potentially inhibit the propagation of their genotype by causing infertility. Our findings suggest that testis-exclusive genes as leading candidates in the genetic aetiology of male infertility. In general, our results emphasize the importance of mapping the sex-specific genetic architecture of humans in order to better understand the evolutionary constraints acting on these genes. This information will facilitate our ability to discover new candidate genes and mutations that may underlie the molecular basis of human disorders. Identification of tissue-specific expression Human gene expression data were taken from the GNF1B oligonucleotide array—the 79 normal tissues and 44,717 gene probes [20] . The Illumina Body-Map RNA-seq 16 human tissue-expression data ( http://www.ebi.ac.uk/arrayexpress/experiments/E-MTAB-513 ) from the GenCards knowledgebase ( http://www.genecards.org/info.shtml#expression_images ) were used for validation. Tissue specificity was calculated by the Pearson correlation coefficient, r [47] , between the gene expression vectors and a synthetic expression vector (mask) of exclusive expression in one tissue, or to any desired expression pattern (for example, giving a value of 0 for non-expressing tissues and a value of 1,000 for the exclusively expressing tissue/s). The masks for the testes included all the combinations of this tissue and the four cell types in it (‘germ cells’, ‘interstitial’, ‘Leydig cells’ and ‘seminiferous tubule’), which are present in the GNF1B data set. Genes with values of 1.0≥ r >0.95 to a mask were considered to have exclusive expression in the expressed tissue/s of that mask. We used the same parameters to identify other non-testis tissue-exclusive genes. Other than the testes, 13 tissues with at least 20 exclusive genes were found and further analysed. These did not include any female-specific tissue (only one exclusive gene found in the ovaries). Finally, in the same way, values of 0.75≥ r >0.65 defined highly specific expression, values of 0.45≥ r >0.35 defined moderate specific expression and values of 0.11≥ r >0.09 defined nonspecific expression for expressed tissue/s of the mask. To avoid redundancy, genes were assigned to a specific group according to their highest r -score. We also excluded genes with transcript isoforms that had different expression patterns in the GNF1B data and genes that had several probe sets. Finally, the GNF1B data results were validated by performing the same expression analysis on the Body-Map data that examined expression in the testes and in 13 other tissues. In comparison with a testis-exclusive mask, 94/95 of our testis-exclusive genes were found in the Body-Map data: 90/94 of these genes have r >0.9, 1 gene has r =0.85, one gene had r =0.77, one gene had r =0.71 and one gene had r =0.48. This last one notable difference was in gene RTKN2 that had an overall low expression in the Body-Map data but was exclusively overexpressed in testis germ cells (but not in whole testes) in GNF1B data. The testis germ cells (and the three other testis cell types) were not represented in the Body-Map data, which might explain this one notable difference from GNF1B data. Identification of male testis-exclusive gene paralogues and male reproduction genes Paralogues for the 95 testis-exclusive genes were retrieved from the GeneCards ( http://www.genecards.org ) human gene compendium [48] . To ascertain that none of these paralogues were not themselves exclusive to the testes, any of these paralogues with r >0.7 with a testis-exclusive-expression mask was excluded from the paralogue list. Male reproduction genes were identified using the Gene Ontology database ( http://www.geneontology.org/ ), searching for human genes under the term ‘Human male gamete formation’, GO:0048232 (which includes all the GO terms enriched in our group of testis-exclusive genes; Table 1 ). Gene data For each analysed human gene, we retrieved the following data from the Ensembl knowledgebase version 69 (release October 2012 to January 2013) using its PERL Application Programming Interface (API) or WWW interface [49] . Data for each gene included its total coding length, and all the variations in the coding regions and four non-coding flank bases of each splice site. Data for each variation included its minor allele count and MAF and total counts of the gene alleles in the ‘1000 Genomes’ project [21] phase-1 data, genomic evolutionary rate profiling evolutionary conservation score, GERP [22] , for mammals and the variation transcription consequence (non-synonymous predicted deleterious, non-synonymous other, stop-gain (nonsense mutations, that is, causing early stop codons), frameshift, splice-site change, transcript ablation, synonymous and others). For all tissue-exclusive genes the protein-coding genes mouse–human dN/dS values were also retrieved. A non-synonymous variation was considered predicted deleterious (pdNS) only when both SIFT [50] and Polyphen [51] methods predicted it as deleterious. A variation can have several transcription consequences for genes with multiple transcripts (for example, the variation can be either synonymous or non-synonymous if its position is in a different translation frame in different transcripts). In such cases the more disruptive outcome to the protein product was considered (that is, pdNS>stop-gain>other-NS>synonymous). The ‘1000 Genomes’ project phase-1 data include 1,092 individuals, and hence 2,184 autosomal alleles for sites present in all individuals. Assuming that the individuals are unrelated to one another, the variation frequency resolution in these data requires two or more observations. For autosomal chromosomes, this is about 1/1,000 (2/2,184). A variation observed only once (1/2,184) has a frequency of about 1/2,000 or less , since it might be less frequent (in an extreme case the variation might only occur in that individual). Random control trial All 20,336 non-Y-linked unique protein-coding human genes listed in the Ensembl knowledgebase version 69 were used to create 10,000 random sets for each tissue-exclusive gene group. The number of genes in each set was the number of genes in the examined gene group. Statistics Comparing testis-exclusive gene groups to the random control sets, we performed a randomization test. The distribution of pdNS accumulation tendencies of all 10,000 random gene sets and the probability of finding the testes pdNS rate randomly were calculated followed by an FDR correction to the different MAF range comparisons. In the same manner a randomization test was performed for each of the other 13 tissue-exclusive gene groups with MAF≥0.005. Since we tested for directional differences (that is, higher than control), when comparing the pdNS tendency of the testis-exclusive genes with that of the non-testis tissue-exclusive gene groups, the testis-exclusive gene paralogues, testis or non-testis tissue specificity groups, we performed a one-tailed case–control χ 2 test. To evaluate the significance of the stop-gain tendency of each of the tissue-exclusive gene groups with that of the non-testis tissue-exclusive genes, we performed a one-tailed binomial exact test. Multiple testing corrections were carried out using Benjamini FDR corrections. The d N /d S distribution test between testis-exclusive genes and the non-testis tissue-exclusive gene groups was evaluated using the KS test. GERP conservation score distribution comparisons of the testis-exclusive genes to their paralogues, to non-testis tissue-exclusive genes or to non-testis-exclusive male reproduction gene groups were performed using two-tailed KS test followed by FDR correction for multiple tests. How to cite this article: Gershoni, M. and Pietrokovski, S. Reduced selection and accumulation of deleterious mutations in genes exclusively expressed in men. Nat. Commun. 5:4438 doi: 10.1038/ncomms5438 (2014).